Crossover from random three-dimensional avalanches to correlated nano shear bands in metallic glasses When applying mechanical stress to a bulk metallic glass it responds with elastic and/or plastic deformations. A comprehensive microscopic theory for the plasticity of amorphous solids remains an open task. Shear transformation zones consisting of dozens of atoms have been identified as smallest units of deformation. The connexion between local formation of shear transformations zones and the creation of macroscopic shear bands can be made using statistical analysis of stress/energy drops or strain slips during mechanical loading. Numerical work has proposed a power law dependence of those energy drops. Here we present an approach to circumvent the experimental resolution problem using a waiting time analysis. We report on the power law-distributed deformation behaviour and the observation of a crossover in the waiting times statistics. This crossover indicates a transition in the plastic deformation behaviour from three-dimensional random activity to a two-dimensional nano shear band sliding. In recent studies, avalanche dynamics and crackling noise [1] have been proven to be important concepts for the description of plasticity in solid media [2] , [3] , [4] , [5] , [6] . Apart from that, avalanche dynamics are well known to occur in a large number of fundamentally different systems, including stick-slip phenomena like earthquakes, Barkhausen noise owing to the pinning/depinning of magnetic domain walls and martensitic phase transitions to name but a few [7] , [8] , [9] . Despite the variety of systems and the complexity of effects, they all exhibit a power law behaviour in the distribution of the avalanche sizes D ( s ) ∝ s − κ with a critical exponent κ . The occurence of a power law distribution indicates the lack of a characteristic length scale and the system to exhibit self-organized criticality [10] . When exposed to mechanical stress, bulk metallic glasses respond as a viscoplastic material, comprising elastic, anelastic and plastic contributions. In creep experiments, a sudden jump to a constant tensile stress level is exerted and the strain is recorded as a function of time. Whereas the elastic deformation occurs almost instantaneously when the external stress is applied, the creep response depicts the anelastic and plastic contributions. For the serrated flow in bulk metallic glasses, stress drops in the plastic regime of stress-strain characteristics can be attributed to the motion and arrest of single shear bands [11] . They have been shown to occur either with a Gaussian size distribution, showing chaotic behaviour, or to obey a power-law-type size distribution, indicating self-organized criticality [12] , [13] . The arrest and reactivation of so-called shear bands, planar regions of highly-localized shear deformation with a thickness of about 10–200 nm (ref. 14 ), has been discussed as the origin of avalanche dynamics in the serrated flow regime. Such concepts might play an important role also on a smaller length scale. In the picture of microscopic plastic events, like ‘shear transformation zones’ (STZs) as introduced by Argon [15] , stress relaxation is localized in ensembles of about 100 atoms [16] , [17] . Although, in mean field descriptions of viscoplasticity [18] , STZs are often regarded to act independently, it is known that they indeed carry a long-range elastic stress field-like an Eshelby inclusion [19] causing cooperative effects among single plastic events [20] , [21] . Finally, their collective activation is responsible for the emergence of macroscopic shear bands [22] , and hence plasticity and failure. On the length scale of such interacting local plastic rearrangements, avalanche statistics have been studied in theoretical efforts and numerical simulations [2] , [4] , [23] , [24] , [25] , [26] . In this article, we report on our observations of power law-distributed waiting times between instrumentally resolvable, equidistant length values in the macroscopically anelastic creep response recorded by Dynamic Mechanical Analysis (DMA). Despite DMA lacking the resolution for directly recording the slip lengths of single microscopic plastic events, this waiting time analysis presents an approach, which gives insight into the statistic properties of microscopic shear deformation. We first analyse the influences of temperature and applied stress on the waiting time distributions obtained from the creep experiments. We discuss these results in terms of a potential energy landscape (PEL) [27] , [28] , [29] , [30] , [31] , where the applied stress assists the thermal activation of STZs by lowering the energy barrier and hence might also facilitate cooperative shear processes, that is, the propagation of an avalanche. Finally, a crossover between two distinct power law regimes is observed in the waiting time statistics of long-time measurements. We argue that this crossover indicates an exhaustion of random stress-assisted avalanche-like events in three dimensions, which is followed by thermally-activated correlated events like nano shear bands in two dimensions. 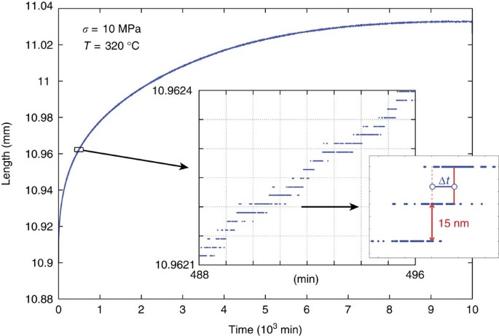Figure 1: Creep curve. A static force was applied to a Pd77.5Cu6.0Si16.5ribbon and held constant for 1 week while recording the sample’s expansion as a function of time. An irregular, step-like deformation behaviour in the microstructure can be observed as visible from the inset wherefore an analysis of waiting times between successive machine resolution steps was motivated. Creep curves Figure 1 shows the long-time expansion behaviour of a Pd 77.5 Cu 6.0 Si 16.5 bulk metallic glass ribbon during a typical creep experiment as described in the methods section. As illustrated in the inset, the machine detects sample length changes with a resolution of 15 nm. Of course, the discreteness of these values does not imply the sample length to actually change in 15 nm steps. Although smaller length changes remain undetected, they do accumulatively contribute to the 15 nm steps. Also note that the creep curve is obviously afflicted with some instrumental noise comprising up and down jumps—we want to emphasize that actual down jumps, that is, a temporary shortening of the sample under applied tensile stress—would be very counterintuitive. Nevertheless, one recognizes at first glance the strain evolution to tread a rather bumpy path. The inset of Fig. 1 shows an aperiodically-alternating behaviour with high and low strain rates instead of a smooth creep curve. Figure 1: Creep curve. A static force was applied to a Pd 77.5 Cu 6.0 Si 16.5 ribbon and held constant for 1 week while recording the sample’s expansion as a function of time. An irregular, step-like deformation behaviour in the microstructure can be observed as visible from the inset wherefore an analysis of waiting times between successive machine resolution steps was motivated. Full size image Since we are unable to investigate the microscopic dynamics of plastic deformation directly by measuring slip lengths, we perform a waiting time analysis by computing the temporal distance Δ t between each pair of successive 15 nm length steps. We set up statistics of waiting times by plotting their frequency of occurence in a histogram. By defining the step positions in the experimental data (see methods section), it is possible to distinguish the actual signal from the underlying machine’s noise. Then the distribution of waiting times can be easily evaluated. Short-time measurements For the short-time measurements the force was kept constant for 180 min and the strain was recorded as a function of time. 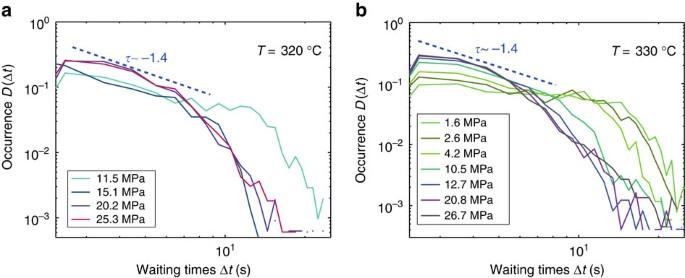Figure 2: Short-time measurements. Waiting time distributions obtained from creep curves at 320 °C (a) and 330 °C (b). A power law behaviour with a stress- and temperature-dependent cutoff is found. Beyond a characteristic stressσc, the cutoff exhibits no further shift. Figure 2 shows the distribution of waiting times for different stresses and temperatures, respectively. At 320 °C, all distributions obey a power law followed by an exponential decay for long waiting times. As illustrated by the trend line, a power law exponent of τ =−1.4 holds for all curves at this temperature. Increasing the stresses up to a characteristic stress σ c , the distributions tend to decay at shorter waiting times. Beyond σ c ≈15 MPa no significant further shift of the cutoff positions is observed. Figure 2: Short-time measurements. Waiting time distributions obtained from creep curves at 320 °C ( a ) and 330 °C ( b ). A power law behaviour with a stress- and temperature-dependent cutoff is found. Beyond a characteristic stress σ c , the cutoff exhibits no further shift. Full size image In addition, the waiting time distributions are sensitive to temperature and tend to exhibit significantly shorter average waiting times when approaching the glass transition temperature. At 330 °C, the characteristic exponent becomes difficult to determine owing to an earlier cutoff, lying still in the neighbourhood of τ =−1.4. The characteristic stress σ c is reduced to ~10 MPa. In addition, we see a form of onset of a plateau for small stresses, delaying the descent of the distribution towards higher waiting times. Long-time measurements We used the same procedure as for the short-time measurements except for applying the creep force for 1 week instead of 180 min. The corresponding experiments were taken at T =320 °C. We see the waiting time distribution for the entire experiment extending towards longer waiting times (see Fig. 3 , grey curve), which simply reflects the contribution from the later part of the creep experiment where the strain increase is continuously slowing down. In contrast to the short-time measurements, no cutoff can be seen as the creep extension slows down and long waiting times gain in statistical weight in the later part of the curve. 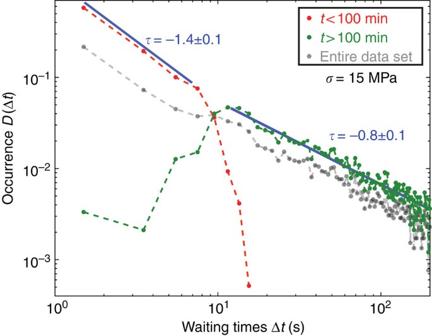Figure 3: Long-time measurements. The waiting time distribution can be split up into two power law regimes with different slopes, originating from the first 100 min of the creep curve and the subsequent part. Figure 3: Long-time measurements. The waiting time distribution can be split up into two power law regimes with different slopes, originating from the first 100 min of the creep curve and the subsequent part. Full size image We finally report on a crossover observable in the waiting time distributions obtained from long-time creep measurements. By looking at the data before and after 100 min experimentation time separately, a crossover is revealed. We observe a transition from a steeper descent ( red curve) to a region declining more flatly ( green curve). The crossover between two distinct power law regimes is illustrated by the trend lines in Fig. 3 . The early part exhibits an exponent of τ (1) =−1.4±0.1—as expected, since it is essentially a short-time measurement. In the second power law regime, which originates from the data recorded after 100 min, the exponent is changed to τ (2) =−0.8±0.1. The algorithm extracting the step positions in time from the experimental data sets gives results where each two successive data points are displaced by 15 nm. The waiting time here is the horizontal interval of the two steps, that is, the time elapsed to reach a constant length change of 15 nm. First, we note that nearly instantaneous elastic deformation is not depicted in our creep curves but has appeared already before. Furthermore, the anelastic regime studied here is far off the region where macroscopic- and system-spanning shear bands appear, both in time and stress. It is known from simulational approaches that correlated STZ activity, that is, inhomogeneous deformation, typically occurs at temperatures below T g and high stresses [23] , [32] . Hence, we attribute the 15 nm length steps to the occurrence of the so-called ‘nano shear bands’. This term expresses the cooperative behaviour of STZs, which arrange in small shear planes, as studied in recent theoretical works [33] , [34] . We want to emphasize again that the restriction to this 15 nm length changes is purely a consequence of the machine resolution. One must of course assume nano shear bands to occur at various sizes. An easy estimation illustrates that a 15 nm length change usually cannot be attributed to a single event only: On the assumption of a typical STZ size of about 1000 atoms or 3.5 nm diameter, which exhibits a length change of 2% (the yield strain), a 15 nm length change would correspond to a simultaneous activation of ≈200 layers of STZs (or ≈300 in form of a shear band oriented 45° towards the stress axis) in a single process. The formation of nano shear bands, where many STZs are cooperatively activated under stress, can be regarded as an avalanche-like process where the activation rate of STZs is significantly enhanced during the avalanche process. Thus, the waiting time is regarded as the time needed to establish a certain amount of nano shear bands in the sample. The observed variations in the waiting time or, analogously, the sometimes-ragged form of the creep curve can then be attributed to a changing activation rate of STZs, that is, avalanche dynamics. According to the PEL model [27] , [28] , [29] , [30] , [31] temperature and stress both may drive the system over barriers. Hence, at a given temperature, the applied stress plays an important role. Only when assisted by the stress, the random thermal activation of STZs might trigger small plastic avalanches in certain directions mediated by short-range interactions [23] . These nano shear bands are created independently and are distributed randomly in the three-dimensional sample. It is known from avalanche simulations that large events come almost to an arrest several times before they finally stop, showing them to be made up of several smaller subavalanches [1] , [35] . In our case, one must take into account that the maximum avalanche size is probably confined by the inhomogeneous mechanical properties of Pd 77.5 Cu 6.0 Si 16.5 , as seen in elasticity maps, where spatial distributions of the elastic moduli have been found on a nanometre scale [21] , [36] , [37] . With increasing stresses, larger avalanches are initiated and the activation rate of STZs is increased—therefore the probability of long waiting times gets reduced. However, the cutoff revealed in the short-time measurements cannot be ascribed to a complete extinction of long waiting times as we see a continuation of the power law regime in the long-time measurements at identical experimental conditions. This indicates the cutoff to have its origin primarily in the temporal restriction of the short-time experiment. Qualitatively, it can be related to stress-dependent cutoffs as observed in the slip length distributions in other works [1] , [2] . This comparison agrees in particular with the observed shift behaviour of the cutoff position and its saturation at the characteristic stress σ c (see Fig. 2 ). Approaching this stress, the cutoff in avalanche size distributions vanishes as system-spanning events set in ref. 2 . Intuitively, just the opposite must hold for waiting times, where the cutoff becomes more significant for increasing stresses because the stress-driven cascading activation of STZs proceeds more rapidly. Before the crossover, at σ c , an avalanche does not come to an arrest before having formed the largest uncorrelated shear event possible. These independent processes determine the cutoff position and no further shift is expected. Increasing temperature, the system can explore the PEL more easily and, hence, the formation of even larger avalanches is facilitated. This assumption is in good agreement with the experimentally observed earlier cutoff and lower σ c (see Fig. 2 ). The crossover to another power-law-type distribution in the long-time experiments indicates an exhaustion of the mechanical stimulation of these three-dimensionally uncorrelated nano shear bands. The short-time regime, where the mechanical stress assists STZ activation owing to short-range cooperativity among STZs, is followed by a regime dominated by stochastic thermal activation of such STZs that are not able to cause an additional avalanche in their environment. Nevertheless, the increased density of preformed nano shear bands might still lead to long-scale cooperative behaviour among them for even longer times or at higher stresses and ultimately result in the formation and motion of macroscopic shear bands. We hence ascribe the ongoing anelastic deformation in the long-time regime to the cooperative motion of a percolative network of preexisting nano shear bands. Collective stick-slip-like processes might explain why the long-time behaviour still exhibits avalanche dynamics, but now with a different characteristic power law exponent. This cooperative motion is a typical two-dimensional process, which continues the deformation via thermal activation. To conclude, the experimental data agrees with the assumption of a crossover from an uncorrelated nano shear band regime, formed by the stress-assisted short range cooperativity of STZs, to a regime dominated by collective nano shear band activity. In the first regime, large but three-dimensionally uncorrelated clusters are frequently created in avalanche-like events. Their size distribution determines the extension behaviour and its statistical properties. The observed crossover reflects an exhaustion in the formation of such nano shear bands. The subsequent slow long-time creep behaviour is owing mainly to thermally-activated cooperative motion, a two-dimensional process localized in a network of preformed nano shear bands. Sample preparation The measurements were performed on ribbons of a Pd 77.5 Cu 6.0 Si 16.5 metallic glass composition fabricated using arc-melting procedure followed by melt-spinning method. The ribbons' thicknesses are about 40 μm whereby this value can vary within one batch. The glass transition temperature of the Pd 77.5 Cu 6.0 Si 16.5 samples is located at 340 °C. DMA creep measurements For the experimental procedure the samples were mounted on two aluminium holders on either side and then clamped into a PerkinElmer DMA 7. A small pre-stress of 1–1.5 MPa was applied to keep the ribbons stable while heating them up to temperatures between 320 and 330 °C at a heating rate of 40 K min −1 . Then the mode was switched to creep at a certain force for 180 min or 9999, min (short-time and long-time experiments), respectively. By applying the force a corresponding tensile stress is induced on the sample. The DMA 7 is located inside a glove box to avoid contamination of the sample. Waiting time analysis As shown in Fig. 1 machine noise and resolution create the demand for an algorithm, which defines single length/time pairs for each 15 nm step in the data set. We first collect the temporal occurences of each length value into a separate data set. As sample contractions appear unreasonable under applied tensile stress, we assume a monotonic increase of strain-overlapping data sets ascribed to the machine noise. To detect the exact step positions for such overlaps, the algorithm compares the percentages of data points before and after the step positions for both data sets. In detail, the step positions are assigned to that specific time value when, for the first time, less data points are remaining from the upcoming step than data points have passed from the preceding step. The waiting times studied throughout this report correspond to the time intervals between such step positions. The errors bars for the exponents were estimated by 95% confidence intervals. How to cite this article: Krisponeit, J.-O. et al . Crossover from random three-dimensional avalanches to correlated nano shear bands in metallic glasses. Nat. Commun. 5:3616 doi: 10.1038/ncomms4616 (2014).